Corals record long-term Leeuwin current variability including Ningaloo Niño/Niña since 1795 Variability of the Leeuwin current (LC) off Western Australia is a footprint of interannual and decadal climate variations in the tropical Indo-Pacific. La Niña events often result in a strengthened LC, high coastal sea levels and unusually warm sea surface temperatures (SSTs), termed Ningaloo Niño. The rarity of such extreme events and the response of the southeastern Indian Ocean to regional and remote climate forcing are poorly understood owing to the lack of long-term records. Here we use well-replicated coral SST records from within the path of the LC, together with a reconstruction of the El Niño-Southern Oscillation to hindcast historical SST and LC strength from 1795 to 2010. We show that interannual and decadal variations in SST and LC strength characterized the past 215 years and that the most extreme sea level and SST anomalies occurred post 1980. These recent events were unprecedented in severity and are likely aided by accelerated global ocean warming and sea-level rise. The Leeuwin current (LC) transports warm, low-salinity tropical waters southwards along the western coast of Australia, and is the lifeline for diverse and unique tropical-temperate marine ecosystems [1] , [2] , [3] ( Fig. 1a ). El Niño-Southern Oscillation (ENSO) events are known to be one of the major drivers of interannual variations in LC strength through their modulation of equatorial western Pacific zonal wind-stress (WPZWS) anomalies [4] . Through the coastal waveguide, these wind-stress anomalies, in turn, drive changes in the interannual sea level and hence LC strength, and sea surface temperature (SST) anomalies along the coast of western Australia (WA) [1] , [4] . La Niña events are associated with a stronger than normal LC and warm SST anomalies [2] . The latest 2010/11 La Niña event led to unprecedented warming offshore WA, the so-called ‘Ningaloo Niño’ [4] , and the first ever reports of large-scale coral bleaching and fish kills [2] , [3] , [4] . The magnitude of this warming event was enhanced by the multi-decadal warming trends in the western Pacific, strong preceding warming in the tropical Indian Ocean in 2010 (ref. 4 ) and a negative Indian Ocean Dipole [5] . 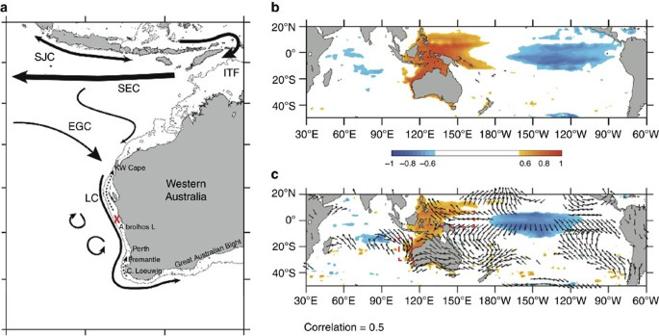Figure 1: Regional surface ocean properties in the Indo-Pacific. (a) Regional surface ocean currents in the eastern Indian Ocean (modified after7). ITF, Indonesian throughflow; SJC, South Java Current; SEC, South Equatorial Current; EGC, East Gyral Current; LC, Leeuwin Current; dotted arrows, inshore currents. The 200 m isobath of bottom topography is shown as solid line. The X (red) indicates the location of the Houtman Abrolhos Islands. Fremantle is indicated where the sea-level station record was established. (b) Spatial correlation of annual Fremantle sea level (FSL) with global sea surface height (SSH) from Simple Ocean Data Assimilation (SODA) 2.0.4 (ref.40) for the calendar year January–December for 1981–2010. (c) Houtman Abrolhos Islands (HAI) regional SST spatial correlation with global sea surface height (SSH, in colour) from SODA 2.0.4 (ref.40), and zonal/meridional wind speed and vectors from twentieth century reanalysis22(arrows proportional to correlation with HAI SST). The rectangular box (stippled red) in the West Pacific called WPZW incindicates the area where Western Pacific Zonal wind stress (3°S-3°N, 130–160°E) is highly correlated with HAI OI SST. The box off WA (stippled red) incshows the location of meridional wind changes (MW WA, 20–30°S, 110–116°E) of importance for HAI SST. Arrows incpoint to dominant wind direction for wind speed anomalies. Only correlations withP<0.05 are shown in colour. Correlations computed athttp://climexp.knmi.nl41. Figure 1: Regional surface ocean properties in the Indo-Pacific. ( a ) Regional surface ocean currents in the eastern Indian Ocean (modified after [7] ). ITF, Indonesian throughflow; SJC, South Java Current; SEC, South Equatorial Current; EGC, East Gyral Current; LC, Leeuwin Current; dotted arrows, inshore currents. The 200 m isobath of bottom topography is shown as solid line. The X (red) indicates the location of the Houtman Abrolhos Islands. Fremantle is indicated where the sea-level station record was established. ( b ) Spatial correlation of annual Fremantle sea level (FSL) with global sea surface height (SSH) from Simple Ocean Data Assimilation (SODA) 2.0.4 (ref. 40 ) for the calendar year January–December for 1981–2010. ( c ) Houtman Abrolhos Islands (HAI) regional SST spatial correlation with global sea surface height (SSH, in colour) from SODA 2.0.4 (ref. 40 ), and zonal/meridional wind speed and vectors from twentieth century reanalysis [22] (arrows proportional to correlation with HAI SST). The rectangular box (stippled red) in the West Pacific called WPZW in c indicates the area where Western Pacific Zonal wind stress (3°S-3°N, 130–160°E) is highly correlated with HAI OI SST. The box off WA (stippled red) in c shows the location of meridional wind changes (MW WA, 20–30°S, 110–116°E) of importance for HAI SST. Arrows in c point to dominant wind direction for wind speed anomalies. Only correlations with P <0.05 are shown in colour. Correlations computed at http://climexp.knmi.nl [41] . Full size image There is a significant correlation between the ENSO (Nino3.4 index [6] ) and Fremantle sea level (FSL), a proxy for LC strength, and SST from 1980 to 2010 (ref. 7 ) ( Fig. 1b ). However, the correlation between Nino3.4 (ref. 6 ) and coastal SST before 1980 is weaker ( Supplementary Fig. 1 ). This suggests that, in addition to ENSO, other processes controlling regional SST need to be accounted for to explain the full range of historical sea level (LC strength) and SST anomalies. Besides the equatorial zonal wind anomalies associated with ENSO, LC strength is also modulated, to some extent, by regional eastern Indian Ocean meridional winds ( Fig. 1c ). Regional SST is influenced by local winds in two ways; one is by modulating the LC variability that then drives the SST variations [7] ; the other is by modulating the air-sea heat exchange [4] . However, long records of local winds are scarce. Here we develop a long record of LC SST from coral proxy data that partly reflects the effect of local wind forcing on the LC, and demonstrates that a linear combination with ENSO forcing and local forcing can provide a robust record of LC strength for the past 215 years. Coral paleoclimatic records Coral core samples were obtained from the Houtman Abrolhos Islands (HAIs) in 2010 ( Fig. 1a ). This is a group of carbonate platforms lying ~50–60 km offshore the western coast of WA, and is home to the southernmost true coral reef formations in the southeastern Indian Ocean [8] . The HAIs lie within the path of the LC, and they support an astonishing diversity of corals for such a high-latitude reef [9] (28.5°S, 113°E). Given their latitude, the HAIs are subject to relatively low intra-annual SST variation of ~4 °C. This is largely attributable to the LC, which bathes the islands in warm tropical water even during winter months [10] , [11] . The intra-annual variation in salinity of ~0.4 psu is also low [12] . However, interannual variability of mean annual HAI SST is high, with La Niña years being significantly warmer (annual mean temperature in 2011 was 1.5 °C above the twentieth century average SST) than El Niño years [10] . To overcome limitations of short-term instrumental ocean observations, paleoclimate records were developed from cores extracted from long-lived Porites corals. Coral δ 18 O and Sr/Ca are widely used as robust proxies for SST [13] , [14] , [15] . While Sr/Ca is considered to be primarily controlled by SST, coral δ 18 O can be influenced by both SST and δ 18 O seawater variations through precipitation minus evaporation (P−E) influencing surface ocean salinity [15] , [16] . However, interannual changes in P−E at the HAIs [12] are too small to noticeably affect coral δ 18 O. Therefore, we assume the δ 18 O record reflects primarily variations in SST. We combine a previously published bimonthly resolved coral δ 18 O record [12] with three new annually resolved Sr/Ca and δ 18 O records to reconstruct a robust record of past SST variability in the LC. Kuhnert et al. [12] made a first attempt to link coral δ 18 O to LC variability using sea-level data from Geraldton (WA) based on spectral analysis of a single core, and found only weak correlations. Here, we used a well-replicated data set and two established coral SST proxies to reconstruct past FSL (a proxy for LC variability), accounting for the influence of the regional wind field and ENSO on the LC. SST reconstruction In this study a 215-year record of reconstructed mean annual SST is derived from coral δ 18 O and/or Sr/Ca variations in three cores from the HAIs ( Figs 1a , 2a–c ; Supplementary Figs 2–5 ; Supplementary Tables 1 and 2 ). In brief, we first, normalized (subtract mean and divide by s.d.) each individual coral record to its variance using the time period 1900–1993 shared by all cores; second, aligned the new annually resolved Sr/Ca and δ 18 O records with the Kuhnert et al. [12] annual time series, and third, averaged all records to form a composite chronology that extends from 1795 to 2010. We converted our normalized coral composite proxy record to SST by scaling it to the s.d. of extended reconstructed SST (ERSST)v3b [17] (over the period 1900–1993), the longest continuous SST data set for the HAI region ( Fig. 2a ; Supplementary Fig. 5 ). The reconstructed mean annual SST was verified against three SST data sets: (1) the NOAA 0.25° × 0.25° gridded Advanced Very High-Resolution Radiometre Optimally Interpolated SST (AVHRR OISSTv2 (ref. 18 ); 28°S, 114°E), (2) the 2° × 2° (27–29°S, 112–114°E) gridded ERSST from NOAA version 3b [17] and (3) the 5° × 5° (25–30°S, 110–115°E) gridded HadSST3 from the Hadley Centre in the UK [19] ( Supplementary Tables 1, 3 and 4 ). 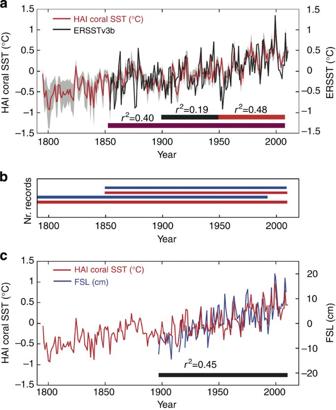Figure 2: Houtman Abrolhos Islands coral composite SST reconstruction from 1795 to 2010. (a) Reconstructed HAI coral SST (red) compared with regional SST from gridded ERSSTv3b17(black) and squared correlation coefficients (P<0.001) indicated for sub-periods. SST anomalies computed relative to the 1900–1993 mean. Coral-derived SST anomalies were scaled by the s.d. of ERSSTv3b17over the same period (1σ=0.37 °C). The two s.e. is indicated for the HAI coral SST (grey shading), (b) number of coral records (blue=δ18O; red=Sr/Ca) and (c) Reconstructed HAI coral SST (red) versus observed Fremantle sea-level (FSL; blue) with squared correlation coefficients indicated. Figure 2: Houtman Abrolhos Islands coral composite SST reconstruction from 1795 to 2010. ( a ) Reconstructed HAI coral SST (red) compared with regional SST from gridded ERSSTv3b [17] (black) and squared correlation coefficients ( P <0.001) indicated for sub-periods. SST anomalies computed relative to the 1900–1993 mean. Coral-derived SST anomalies were scaled by the s.d. of ERSSTv3b [17] over the same period (1 σ =0.37 °C). The two s.e. is indicated for the HAI coral SST (grey shading), ( b ) number of coral records (blue=δ 18 O; red=Sr/Ca) and ( c ) Reconstructed HAI coral SST (red) versus observed Fremantle sea-level (FSL; blue) with squared correlation coefficients indicated. 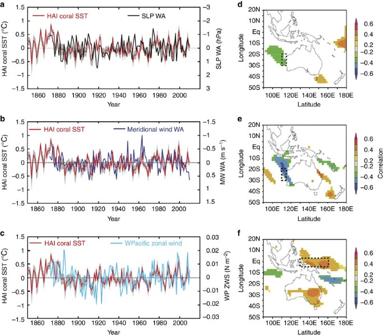Figure 3: Regional and remote wind forcing of HAI SST. Detrended HAI coral SST (red) with two s.e. (grey shading) compared with (a) sea-level pressure off Western Australia (SLP WA, black), (b) meridional wind off Western Australia (MW WA, blue) and (c) Western Pacific zonal wind stress (WPZWS; light blue), all from twentieth century reanalysis22. Spatial correlation of HAI coral composite SST with (d) sea-level pressure with stippled black box off WA, (e) meridional wind with stippled black box off WA showing the location of meridional wind changes of importance for HAI SST and (f) zonal wind stress with stippled rectangular box, WPZWS, indicating the area where Western Pacific Zonal wind stress is highly correlated with HAI SST, all from twentieth century reanalysis for 1960–2010 averaged between January and December for 3dande, and for July to June for 3f. Only correlations withP<0.05 are shown in colour. All time series were detrended and correlation maps computed athttp://climexp.knmi.nl41. Full size image For the non-detrended data, a significant correlation ( r =0.65, P <0.001) was found between reconstructed SST and AVHRR OISST for the period from 1981 to 2010 ( Supplementary Table 3 ). We also found significant correlations with ERSST ( r =0.63, P <0.001) and HadSST3 ( r =0.66, P <0.001) between 1960 and 2010, the period in which the observational data coverage is acceptable in this region. Correlations also remained statistically significant when the series were extended back to the 1850s ( r =0.63, P <0.001 with ERSST; r =0.66, P <0.001 with HadSST3 since 1870; Fig. 2a ; Supplementary Fig. 5 ). 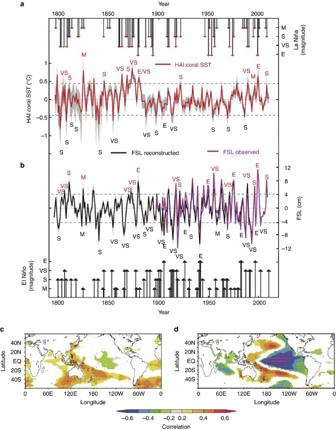Figure 4: Detrended HAI coral SST and Fremantle sea-level. (a) Detrended HAI coral SST reconstruction (red line with two s.e. as grey shading; ±1σs.d.=grey dashed lines), (b) fremantle sea-level (FSL) observations (purple line) and FSL reconstructed (black line with two s.e. as grey shading; ±1σs.d.=grey dashed lines) based on linear model including PC1 of Kuhnertet al.12January–June coral record and paleo-ENSO reconstruction from Wilsonet al.21La Niña and El Niño event magnitude for M, moderate, S, strong, VS, very strong and E, extreme events following Gergis and Fowler23classification indicated above (a) and below (b), respectively. La Niña (red) and El Niño (black) event magnitude indicated by strings for years in (a) and (b) that are above ±1σs.d., (c) spatial correlation of detrended HAI coral SST reconstruction with ERSSTv3b17and (d) spatial correlation of detrended FSL reconstructed (1994–2010 from FSL observations) with ERSSTv3b17. Only correlations withP<0.05 are shown in colour in (c) and (d). Correlations computed athttp://climexp.knmi.nl41. Correlations were statistically significant after detrending, although they are of lower magnitude ( Supplementary Table 4 ). Lower correlations with SST products were generally found between 1900 and 1950 ( Fig. 2a ). There are four possible reasons for this: first, sparser ship-based SST observations in the HAI region affected SST data quality; second, SST data spatial resolution does not resolve reef-scale SST; third, heterogeneity of local reef-scale SST across the HAI coral core sites [10] or forth, growth rate differences between coral cores could have potentially influenced coral SST proxies to a varying extent ( Supplementary Table 2 ). The latter influence cannot be excluded, yet our multi-core, multi-proxy approach was designed to minimize these effects. Given the extremely sparse in situ SST coverage in the region before ~1900 ( Supplementary Fig. 6 ) and the degree of coral core replication in this study, our new proxy-based SST reconstruction probably provides the best estimates of SST for the HAI for this early instrumental period. Our new coral composite SST record shows a linear warming trend of 1.16±0.06 °C (0.054 °C per decade) between 1795 and 2010 ( Fig. 2a ). For the period from 1854 to 2010, which overlaps with the instrumental records, the linear trend in the coral composite SST was +0.76±0.06 °C (0.049 °C per decade), in close agreement with +0.72±0.10 °C (0.046 °C per decade) from ERSST. The linear warming trend after 1950 accounts for most of the long-term warming in both the coral composite and ERSST with values of 0.58±0.10 °C (0.098 °C per decade) and 0.72±0.16 °C (0.117 °C per decade), respectively. A linear warming trend of 0.40 °C (0.066 °C per decade) in coral SST is recorded between 1795 and 1854, predating available ship-based SST observations. This warming follows a series of cool anomalies between 1795 to the mid-1830s coinciding with major volcanic events [20] . Sea-level reconstruction and LC strength HAI AVHRR OISST [18] reveals a close connection with ENSO and downstream FSL anomalies [3] as evidenced by the typical spatial correlation pattern across the tropical Pacific ( Fig. 1b,c ; Supplementary Figs 1 and 2 ; Supplementary Tables 1 and 4 ). Correlation maps of our detrended coral composite SST versus global sea-level height also showed a significant relationship with western Pacific and coastal sea level off WA ( Supplementary Fig. 2 ). FSL data from the long-term tide gauge reference station are the best direct observational records of past LC strength and its relationship with Pacific climate variability [1] ( Fig. 2c ). The data set provides a nearly continuous record from 1943 to the present with intermittent measurements back to 1897. It shows a rising trend in sea level of 1.5 mm per year over the twentieth century associated with global sea-level rise [4] ( Fig. 2c ). Our new, non-detrended coral HAI SST reconstruction is significantly correlated with FSL ( r =0.67, P <0.001) between 1897 and 2010. To reconstruct a 215-year proxy record of the interannual and decadal variations in LC strength (FSL), we first established whether our detrended HAI coral SST record was indeed related to regional wind forcing, and second, that a linear combination with a paleo-ENSO [21] record can provide a robust long-term record of LC strength. We used the twentieth century reanalysis [22] sea-level pressure (SLP), meridional and zonal winds from 1870 to assess the long-term relationship between WPZWS and meridional wind off WA (MWWA) with FSL and HAI SST ( Fig. 3a–c ). We found a significant negative correlation between both instrumental and reconstructed SST with MWWA and SLP (positive with WPZWS) for annual means and in austral summer/autumn ( Fig. 3d–f ; Supplementary Fig. 7 ). Weaker southerly winds off the WA coast are associated with an offshore low SLP center ( Fig. 3d ). This, in combination with easterly zonal winds in the Western Pacific, favours southward transport of warm waters from the northwest Australian shelf via the LC in austral summer/autumn ( Fig. 3e ). A strong relationship between MWWA and the first principal component (hereafter PC1) of bimonthly January–June coral data from Kuhnert et al. [12] was identified ( Supplementary Fig. 7 ). This highlights the importance of the austral summer/autumn response in HAI SST to meridional wind forcing. Having established that regional HAI SST are linked to eastern Indian Ocean meridional winds and SLP off WA, and that MWWA influences FSL, we propose that an accurate reconstruction of FSL (as a proxy for LC strength) can be produced using a linear combination of ENSO forcing and coral proxy-derived SST/wind forcing. Figure 3: Regional and remote wind forcing of HAI SST. Detrended HAI coral SST (red) with two s.e. (grey shading) compared with ( a ) sea-level pressure off Western Australia (SLP WA, black), ( b ) meridional wind off Western Australia (MW WA, blue) and ( c ) Western Pacific zonal wind stress (WPZWS; light blue), all from twentieth century reanalysis [22] . Spatial correlation of HAI coral composite SST with ( d ) sea-level pressure with stippled black box off WA, ( e ) meridional wind with stippled black box off WA showing the location of meridional wind changes of importance for HAI SST and ( f ) zonal wind stress with stippled rectangular box, WPZWS, indicating the area where Western Pacific Zonal wind stress is highly correlated with HAI SST, all from twentieth century reanalysis for 1960–2010 averaged between January and December for 3 d and e , and for July to June for 3 f . Only correlations with P <0.05 are shown in colour. All time series were detrended and correlation maps computed at http://climexp.knmi.nl [41] . Full size image We used a linear regression model that takes into account the remote forcing from ENSO variability based on various ENSO indices and the regional SST at HAI (detrended) at either annual resolution (calendar year January–December), using the coral composite SST, or focusing on the summer/autumn period by using PC1 (January–June) of the bimonthly coral δ 18 O Kuhnert et al. [12] data to reconstruct annual mean FSL ( Supplementary Fig. 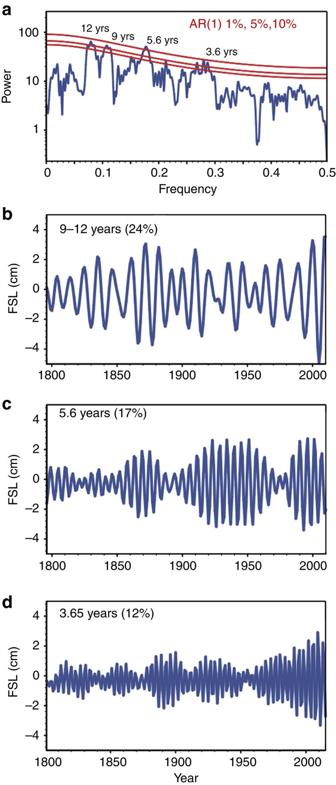Figure 5: Spectral analysis of the FSL reconstruction and dominant frequencies. (a) Multi-taper spectrum of reconstructed FSL (1795–1993) based on linear model with PC1 of Kuhnertet al.12and reconstructed ENSO index (COA) of Wilsonet al.21combined with observed FSL (1994–2010). The mean frequency of the main bands is indicated. Confidence levels for 10, 5 and 1% are indicated as red lines with the upper line being the 1% level. (b–d) Reconstructed components of the FSL reconstruction with years from 1994 to 2010 based on observed FSL. All frequencies withP<0.05. Explained variance indicated in brackets. (b) 9–12 year, (c) 5.6 year and (d) 3.65 year frequency. 7 ; Supplementary Table 5 ). We tested a set of paleo-ENSO indices that extend before 1854 as covariates in the linear model. The best model included PC1 of the Kuhnert et al. [12] data in combination with the Wilson et al. [21] paleo-ENSO index (for the region in the central and eastern Pacific) for the period 1795–1993. The model explained 74% ( P <0.001) of variance in FSL for the calibration period, 1950–1993, and 64% of variance in FSL ( P <0.001) for the independent verification period, 1924–1949 ( Supplementary Table 5 ). The paleo-ENSO index alone explained 62% ( P <0.001) of variance in FSL for the calibration period, 1950–1993, and 47% of variance in FSL ( P <0.001) for the verification period, 1924–1949. Given this stability of the relationships, we reconstructed variations in annual mean FSL (reflecting LC strength) back to 1795 ( Fig. 4b ; Supplementary Fig. 8 ). Figure 4: Detrended HAI coral SST and Fremantle sea-level. ( a ) Detrended HAI coral SST reconstruction (red line with two s.e. as grey shading; ±1 σ s.d.=grey dashed lines), ( b ) fremantle sea-level (FSL) observations (purple line) and FSL reconstructed (black line with two s.e. as grey shading; ±1 σ s.d.=grey dashed lines) based on linear model including PC1 of Kuhnert et al. [12] January–June coral record and paleo-ENSO reconstruction from Wilson et al. [21] La Niña and El Niño event magnitude for M, moderate, S, strong, VS, very strong and E, extreme events following Gergis and Fowler [23] classification indicated above ( a ) and below ( b ), respectively. La Niña (red) and El Niño (black) event magnitude indicated by strings for years in ( a ) and ( b ) that are above ±1 σ s.d., ( c ) spatial correlation of detrended HAI coral SST reconstruction with ERSSTv3b [17] and ( d ) spatial correlation of detrended FSL reconstructed (1994–2010 from FSL observations) with ERSSTv3b [17] . Only correlations with P <0.05 are shown in colour in ( c ) and ( d ). Correlations computed at http://climexp.knmi.nl [41] . Full size image Positive reconstructed FSL anomalies occur at major La Niña events, while negative anomalies occurred during major El Niño years (based on the ENSO event classification of Gergis and Fowler [23] ( Fig. 4a–d ). The period between 1800 and 1811 showed large positive FSL anomalies, with 1810/11 being the highest, in line with the occurrence of a series of strong La Niña events and very wet conditions in north-east Australia [23] , [24] ( Fig. 4b ; Supplementary Fig. 8 ). The period between 1820 and 1860 showed reduced interannual variability in LC strength ( Fig. 5c ). Between 1860 and 1885, LC interannual variability increased, leading to the largest FSL fluctuations pre-1900 with the 1879/80 La Niña having the highest and 1865/66 El Niño the lowest FSL anomalies ( Fig. 5c ). Between 1900 and 1960, interannual variability remained high with 1909/10, 1917, 1934, 1945, 1950 and 1955/56 showing higher sea levels during La Niña’s. From 1960 through the mid-1990s, decadal LC variability persisted superimposed on a general weakening trend ( Fig. 5b ). The strongest interannual events occurred in 1962/63, 1971, 1974/75 and 1989, all La Niña events. After 1995, LC strength from the observational record showed a decadal strengthening and large positive FSL anomalies marked the intense La Niña events in 1996, 1999 and 2008. Figure 5: Spectral analysis of the FSL reconstruction and dominant frequencies. ( a ) Multi-taper spectrum of reconstructed FSL (1795–1993) based on linear model with PC1 of Kuhnert et al. [12] and reconstructed ENSO index (COA) of Wilson et al. [21] combined with observed FSL (1994–2010). The mean frequency of the main bands is indicated. Confidence levels for 10, 5 and 1% are indicated as red lines with the upper line being the 1% level. ( b – d ) Reconstructed components of the FSL reconstruction with years from 1994 to 2010 based on observed FSL. All frequencies with P <0.05. Explained variance indicated in brackets. ( b ) 9–12 year, ( c ) 5.6 year and ( d ) 3.65 year frequency. Full size image Interannual and decadal FSL (LC) variability are persistent features during the 19th and 20th centuries off the west coast of Australia ( Figs 4b and 5c ). Spectral analysis of reconstructed FSL using the Multi-taper method showed significant periodicities at 9–12, 5.6 and 3.65 years ( Fig. 5a ). Those frequncies are typically associated with interannual and decadal ENSO variability [6] , [23] . Variability at 9–12 years persisted for the entire 215 years with strongest amplitudes between 1830s and 1840s, 1860 and 1885, 1910s and after the 1990s ( Fig. 5b ; Supplementary Fig. 6 ). The strongest interannual variability in the 3.65 and 5.6 year bands occurred during the twentieth century, considerably higher in magnitude than for the nineteenth century ( Fig. 5c ; Supplementary Fig. 6 ). We assessed the stability of the relationship between observed FSL, reconstructed FSL and HAI SST for the past 215 years ( Supplementary Fig. 9 ). We find that the magnitudes of HAI SST anomalies are not simply related to LC strength. This is most apparent for the mid-to-late nineteenth century ( Supplementary Fig. 9 ). This indicates that meridional winds (through air-sea heat flux) and SLP off WA and remote forcing of the LC by WPZWS (through advection) played an important role in determining the magnitude of SST anomalies [4] , especially for La Niña and El Niño events. This is illustrated for the past 140 years using the twentieth century reanalysis data of zonal and meridional winds and SLP in comparison with HAI SST and observed/reconstructed FSL ( Figs 3a–f and 4a,b ; Supplementary Figs 9 and 10 ). The spatial distribution of the correlation with reconstructed FSL also showed a much stronger ENSO teleconnection pattern with Indo-Pacific SST than local HAI SST ( Fig. 4c,d ; Supplementary Figs 11 and 12 ). Furthermore, 15-year running correlations revealed that the relationship between HAI coral and instrumental SST with ENSO (Niño-4 index or paleo-ENSO) [6] , [23] was not constant over the past 215 years with higher correlations occurring during periods of stronger La Niña activity ( Supplementary Fig. 1 ). The LC is known to vary on interannual and decadal time scales during the twentieth century, to a large extent driven by ENSO and the Pacific Decadal Oscillation [1] . Lower FSL (detrended) was observed between 1970 and1990, followed by an increase after the early 1990s [25] . Whereas this phase transition was mostly driven by decadal variations in WPZWS [25] , [26] , considerable uncertainty exists around its linkage with long-term climate change [4] . The question also arises as to how future climate change will impact LC strength and SST anomalies in light of such strong decadal variations. The robust paleoclimatological reconstruction of LC strength described here provides long-term insights into the interannual and decadal behaviour of the LC that build on current knowledge of the link between SST and meridional wind off the west coast of Australia, sea level and remote forcing from the Pacific via ENSO and western Pacific zonal wind stress [4] . Our new reconstruction reveals that the magnitude of FSL anomalies during past ENSO events has varied. The twentieth century shows greater FSL interannual variability than the nineteenth century while decadal variability was a persistent feature in both periods ( Fig. 5a–d ). It may be the case that warming of the tropical oceans [27] has intensified the variability of sea level and SST along the WA coast with potential consequent effects on the unique biodiversity of this region. Our HAI coral-based SST reconstruction showed significant warming over the past 215 years, with current SSTs at their highest level since at least 1795 ( Fig. 2a ). High sea-level anomalies generally coincide with marked warming events over the 215-year record ( Fig. 2c ). As an example, both the 1975 and 1999 warm SST anomalies were associated with interdecadal peaks in regional sea-level anomalies, illustrating the importance of decadal-scale changes in LC variability in boosting the amplitude of La Niña-associated SST anomalies off WA. The strong La Niña events between 1800 and 1811, with 1810/11 almost of equal strength as 1974/75, occurred during a period of lower mean SST ( Figs 2a and 4a,b ). The amplitude of the SST anomalies during a particular La Niña event depends on the strength and/or direction of the Western Pacific zonal wind stress and the regional meridional wind strength. Feng et al. [4] first showed the importance of regional wind forcing and heat flux in driving extremes in SST and sea level during the Ningaloo Niño event of 2011 along the west coast of Australia. The local amplification of SST anomalies during so-called Ningaloo Niño (warm) or Niña (cold) events by meridional winds off the west coast of Australia was recently confirmed based on 61 years (1950–2011) of instrumental wind and SST data [28] . Our results indicate that very warm SST in the HAI can result from favourable meridional winds off WA despite not all being La Niña years, as happened for instance in 1875, 1880, 1934, 1955, 1962/63 and 1984 ( Fig. 3b,e ). The eastern Indian Ocean shows a robust long-term warming trend, including the source region of the LC from the Indonesian Throughflow to the northwest Australian shelf where the warm water builds up. The warming trend has significantly altered the absolute magnitude of SST extremes during La Niña and El Niño events. The absolute mean annual SST anomalies during La Niña events after 1980 are significantly higher than those occurring between 1795 and 1979 (+0.64 °C, P <0.05, Mann–Whitney U -test). SSTs during El Niño events normally decrease off West Australia but even these anomalies are well above the twentieth century mean SST after 1980 ( Fig. 2a ). The absolute difference of mean annual SST during El Niño events pre- (1795–1979) and post-1980 is +0.58 °C ( P <0.05, Mann–Whitney U -test). We found an intensification of the correlation between reconstructed HAI SST and ENSO after 1980. This strengthened relationship could be a response to the recent dominance of a La Niña-like trend pattern with positive western Pacific warm pool SST anomalies, especially after the 1990s [29] . The recent strengthening of the HAI SST–La Niña relationship suggests that the continued warming over the twenty-first century is likely to increase the magnitude of extreme ‘Ningaloo Niño’s’. The occurrence of Ningaloo Niño’s depends also on the future trajectories of ENSO, Pacific Decadal Oscillation and Indian Ocean Dipole characteristics, and how they interact with regional meridional wind changes in the eastern Indian Ocean. There is a lack of consensus amongst global climate models as to how these major tropical modes will change with continued global warming [30] , [31] . Regional ocean projections under the future climate scenario A1B simulated a 15% reduction in LC strength towards the end of the twenty-first century [32] . Decadal climate variations such as those we have presented are particularly important for such climate projections for the coming decades. Given that the Ningaloo Niño during the 2010/11 heat wave had a profound impact on a variety of marine biota, a more frequent occurrence of such events, together with projected eastern Indian Ocean warming towards the end of the twenty-first century [32] could potentially increase coral bleaching risk and affect maintenance of the current diverse high-latitude coral reef ecosystem and associated fisheries. Coral core collection and microsampling Coral cores were collected in September 2010 during a research cruise of the RV Solander of the Australian Institute of Marine Science ( Supplementary Figs 1–4 ). Core HAB05B (1.31 m length) and HAB10A (1.29 m length) were obtained from the HAIs. All proxy records are obtained from the East Wallabi island group (113°75′E, 28°46′S) with a maximum distance of 2.8 km between collection sites. Core HAB05B was drilled from a Porites sp. colony growing in 3.5 m water depth, whereas the HAB10A Porites sp. colony was living in 8.5 m depth. Cores were cut parallel to their main growth axis into rectangular slabs 7-mm-thick and X-rayed to reveal annual density banding ( Supplementary Figs 13 and 14 ). Growth rates for the corals were determined by counting annual density bands from the X-ray-positive prints confirmed by counting luminescent bands [33] . X-ray-derived density and luminescence banding on the whole core showed excellent agreement, and thus their combined use enabled the most accurate interpretation of the orientation of the growth axis for both cores. The average growth rate of core HAB05B was 0.52 cm per year, whereas HAB10A growth averaged 0.69 cm per year. The published coral stable oxygen isotope (δ 18 O) of Kuhnert et al. [12] was obtained from a coral core collected in May 1994. The Porites lutea colony was 3.7 m high at a depth of 5 m and had an average growth rate of 1.5 cm per year. Ledges of cores HAB05B and HAB10A were milled into the outer edge of the prepared core slabs using the Zenbot Precision Mill. Ledges were made 5 mm thick by ablating 1 mm off the top and bottom of the core edges to expose a clean surface along the growth axis for sampling. The cores were then repeatedly rinsed with de-ionized water and washed in an ultrasonic bath for 10 min, repeated three times, to remove carbonate powder and any stray particles. The core sections were left to soak overnight in a 1:1 mixed reagent grade sodium hypochlorite (NaOCl) and ultra-purified water (Milli-Q, >18 MΩ cm −1 ) solution to remove the outer tissue layer and any residual organic matter in the skeletal matrix. The cores were retrieved the next day and washed repeatedly in de-ionized water and the ultrasonic bath to remove the bleach solution and subsequently dried in an oven at 40 °C for 24 h. The Zenbot Precision Mill at UWA was used to collect annual samples from both cores. The mill is computer controlled (that is, speed, r.p.m. and x/y/z movement) and was fitted with a 2.5-mm diameter tungsten carbide bit. Annual sampling was undertaken by sampling at 2.5 mm depth evenly along the entire length of each annual density band couplet comprising of a low- and high-density band. Analytical procedures for Sr/Ca and δ 18 O All measurements were carried out on a Thermo Fisher Scientific (Bremen, Germany) X Series II quadrupole inductively coupled plasma mass spectrometer using the standard Xt interface and the plasma screen fitted at the University of Western Australia. Long-term reproducibility (RSD, 2 sigma) derived from repeated analyses of the gravimetrically prepared standard yielded 0.4%, Sr/Ca. The stable oxygen isotope (δ 18 O) ratios in Kuhnert et al. [12] were analysed on a Finnigan MAT 251 mass spectrometer calibrated against NBS-19. They are reported in per mil versus Vienna Pee Dee Belemnite isotope scale (‰ VPDB). Analytical errors of replicate measurements of an internal laboratory standard (Solnhofen limestone) are <±0.07 for δ 18 O. The δ 18 O analyses on the new HAB10A coral record was undertaken at the West Australian Biogeochemistry Centre at the University of WA following the protocol of Paul and Skrzypek [34] . The δ 18 O were analysed using GasBench II coupled with Delta XL Isotope Ratio Mass Spectrometer (Thermo Fisher Scientific). All results were expressed using the standard δ-notation (δ 18 O) and were reported in per mil (‰) after normalization to Vienna Pee Dee Belemnite isotope scale (‰ VPDB). The multi-point normalization was based on three international standards NBS18, NBS19 and L-SVEC, each replicated twice [35] . The analytical uncertainty was lower than ±0.10‰ (1σ) for δ 18 O. The proxy data will be made available through NOAA paleoclimate database ( www.ncdc.noaa.gov/paleo/ ). Proxy data treatment We used the published bimonthly coral δ 18 O record of Kuhnert et al. [12] as our reference coral because the presence of seasonal cycles provided the best age control for all cores. We developed two new annually resolved coral core chronologies for Sr/Ca (cores HAB05B and HAB10A) and measured δ 18 O in one core (HAB10A). The age model of the new corals was determined by assigning 1 year of growth to a couplet of high- and low-density banding in X-ray-positive prints cross-checked with luminescence banding [33] . The high-density bands were equivalent to summer and low density to winter. The coral δ 18 O record of Kuhnert et al. [12] was averaged annually (January–December), and then each individual annually resolved coral proxy record was normalized to its variance relative to the 1900–1993 reference period. We used the COFECHA [36] tool to aid in cross-dating the annual time series. We aligned the new annually resolved Sr/Ca and δ 18 O records (normalized relative to the 1900–1993 reference period) with the Kuhnert et al. [12] annual time series, and averaged all records to form a composite chronology that extends from 1795 to 2010. We also examined each proxy record separately for the correlation with regional SST reconstruction from ERSSTv3b [17] . We converted our normalized coral composite and the individual proxy records to SST by scaling them to the s.d. of ERSSTv3b [17] for the Houtman Abrolhos region (0.366 °C) over the period 1900–1993. To allow for the number of coral records decreasing backwards in time, we calculated the two s.e. for each nest of SST reconstructions starting with two records and ending with the composite record of all four proxy time series. We subsequently spliced the two s.e. series together to show the uncertainty in our SST reconstruction over time. Principal components analysis of the Kuhnert et al. [12] bimonthly δ 18 O data was carried out in R (R Development Core Team 2011) [37] using singular value decomposition. Time series for the January–February, March–April and May–June bins were individually detrended (linearly) before the analysis. Bins were treated as variables and years as observations. The loadings for PC1 were −0.51, −0.66 and −0.56 for January–February, March–April and May–June, respectively. PC1 accounts for 64% of the variance in the data for these bins. PC1 scores for years 1795–1993 were used in the FSL reconstruction. We used the software package R to compute the linear models and for the calibration-verification exercise of reconstructing FSL. Linear combinations of individual coral-based SST reconstructions, PC1 of Kuhnert et al. [12] data, the paleo-ENSO index of Wilson et al. [21] and the observed Nino3.4 index from Kaplan et al. [6] were trialled in formulation of the linear predictor. We used 1950–1993as the calibration period, and 1924–1949as the validation period for the FSL hindcast. Akaike Information Criterion was used to select the best model. The model including PC1 of January–February coral δ 18 O from Kuhnert et al. [12] and the paleo-ENSO of Wilson et al. [21] or observed Nino3.4 (ref. 6 ) index resulted in the best models. Use of the annual coral composite rather than PC1 also performed well, but the amplitudes of FSL anomalies were slightly underestimated. The interannual and decadal variability in the FSL reconstruction was similar when using PC1 or the coral composite with or without Kuhnert et al. [12] data in combination with the paleo-ENSO index [21] or observed Nino3.4 index [6] . Other paleo-ENSO indices [38] , [39] performed well in our linear regression model capturing the interannual and decadal variability in observed FSL, yet did not capture the full magnitude of observed FSL anomalies in our reconstruction. Nevertheless, the stability of interannual and decadal variability using different paleo-ENSO records adds confidence that our FSL reconstruction robustly captures these time scales of variability. We used the Mann–Whitney U -test to test for significant differences ( P <0.05) in mean SST extremes for El Niño and La Niña years pre- and post-1980, following the classification of ENSO event years from Gergis and Fowler [23] . Instrumental data FSL data were obtained from the Permanent Service for Mean Sea Level database: http://www.psmsl.org/data/obtaining/stations/111.php . The FSL data were averaged for January–December to account for the lagged correlation with the ENSO that peaks between February and June in the year following ENSO [4] . For verification of the coral proxy SST records, we used the (1) 0.25° × 0.25° AVHRR OISSTv2 from NOAA [18] , (2) the 2° × 2° gridded ERSST from NOAA (ERSSTv3b [17] ) back to 1854 and (3) the 5° × 5° gridded HadSST3 (ref. 19 ) from the Hadley Centre UK. For Indo-Pacific meridional and zonal winds we used the twentieth century reanalysis data [24] starting from 1870 (ref. 22 ). We obtained the paleo-ENSO index from the compilation by Wilson et al. [21] and the instrumentally observed Nino3.4 index from Kaplan et al. [6] How to cite this article: Zinke, J. et al. Corals record long-term Leeuwin Current variability including Ningaloo Niño/Niña since 1795. Nat. Commun. 5:3607 doi: 10.1038/ncomms4607 (2014).